Measuring single-nanoparticle wetting properties by freeze-fracture shadow-casting cryo-scanning electron microscopy Nanoparticles at fluid interfaces are central to a rapidly increasing range of cutting-edge applications, including drug delivery, uptake through biological membranes, emulsion stabilization and the fabrication of nanocomposites. Understanding nanoscale wetting is a challenging issue, still unresolved for individual nanoparticles, and is essential in designing nanoparticle-building blocks with controlled surface properties. The core information about the structural and thermodynamic properties of particles at fluid interfaces is enclosed in the three-phase contact angle θ . Here we present a novel in situ method, on the basis of freeze-fracture shadow-casting cryo-scanning electron microscopy, that allows the measurement of contact angles of individual nanoparticles with 10 nm diameter, and thus greatly surpasses the current state of the art. We study hydrophilic and hydrophobic, organic and inorganic nanoparticles, demonstrating general applicability to systems of fundamental and applied nanotechnological interest. Significant heterogeneity in the wetting of nanoparticles is observed. Nanoparticles (NPs) at fluid interfaces have an essential role in a vast and rapidly increasing range of novel materials and nanotechnology applications, including drug delivery [1] , uptake through biological membranes [2] , emulsion stabilization [3] and the fabrication of nanocomposites [4] . Investigations on the effect of solid particles at liquid interfaces date back to the seminal work on emulsions by Ramsden [5] and Pickering [6] , but, to date, understanding wetting at the nanoscale remains an open and challenging issue [7] , [8] , still unresolved for individual NPs. Considerable experimental and theoretical efforts have been devoted to the study of micro- and nano-particle adsorption, assembly and dynamics at fluid interfaces [9] , which have significant practical applications in the cosmetics, chemical, food and pharmaceutical industries. Liquid interfaces also offer a particularly well-suited template for the self-assembly of two-dimensional materials from NPs with tailored surface properties [4] , [10] . NPs adsorb and bind at interfaces, but, at the same time, are able to move within the interface to explore the energy landscape determined by their interactions. Several specific interactions are present at the interface [11] that are absent in the bulk and can be exploited to direct the assembly of structures unattainable in bulk [12] , [13] . All the points put forth above are strongly dependent on one key parameter: the particle three-phase contact angle θ . This directly determines the flotation height h of the particle relative to the interface, defining thus the structural, dynamical and thermodynamical properties of interfacial NP assemblies. For θ < π /2 ( Fig. 1a ), most of the particle is immersed in water and it is thus termed hydrophilic, conversely, for θ > π /2 ( Fig. 1b ), the particle is hydrophobic. The binding energy Δ E of a solid particle of radius r at the interface between two fluids with interfacial tension γ 0 can be written as Δ E =− πr 2 γ 0 (1−|cos θ |) 2 (ref. 14 ), excluding line tension contributions. [15] Depending on particle size and wettability, adsorption can be more (Δ E ≈ k B T ) or less (Δ E ≫ k B T ) reversible, with consequences on the equilibrium structure of interfacial assemblies and the kinetics of their formation. Moreover, interparticle interactions, for example, capillary [11] , electrostatic [16] and steric [17] , as well as the viscous drag coefficient on a particle as it moves within the liquid interface [18] , strongly depend on the particle immersion in each phase, that is, on θ . 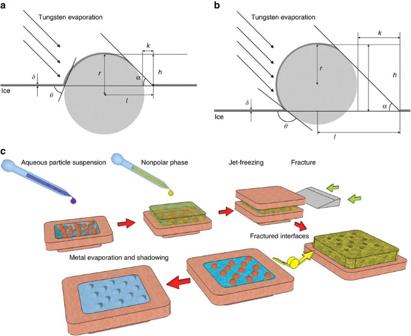Figure 1: Schematics of FreSCa cryo-SEM contact angle measurements. Representation of (a) a hydrophilic and (b) a hydrophobic nanoparticle of radiusrat the ice interface after metal evaporation. The three-phase contact angleθ, the metal deposition angle α and thicknessδ, the heighthof the particle relative to the interface, its projectionlalong the metal deposition direction and the length of the shadowkare highlighted. (c) Scheme of the sample preparation for FreSCa cryo-SEM imaging. Figure 1: Schematics of FreSCa cryo-SEM contact angle measurements. Representation of ( a ) a hydrophilic and ( b ) a hydrophobic nanoparticle of radius r at the ice interface after metal evaporation. The three-phase contact angle θ , the metal deposition angle α and thickness δ , the height h of the particle relative to the interface, its projection l along the metal deposition direction and the length of the shadow k are highlighted. ( c ) Scheme of the sample preparation for FreSCa cryo-SEM imaging. Full size image Unfortunately, the standard use of Young's equation to obtain θ for nanoparticles (cos θ =( γ 2 - γ 1 )/ γ 0 , where γ 1 and γ 2 are the interfacial tensions between the liquid phases and the bulk NP material) often leads to large errors because of several factors that become relevant at the nanoscale; heterogeneity in surface roughness and chemistry have a significant role, and corrections to Young's equation stemming from line tension effects become increasingly more important [11] , [15] . Therefore, several routes have been devised to obtain θ for colloidal particles, either by direct visualization or by inferring it from measurements of global interfacial quantities. The latter typically relies on recording surface pressure/area isotherms in a Langmuir trough [19] , [20] or on measuring the monolayer height relative to the interface using ellipsometry [21] or reflectometry [22] . These techniques can in principle be used for small NPs, but only give an average value without resolving properties on the single-particle level and rely heavily on specific assumptions that are often not applicable. Direct measurements of θ on single particles, for example, by colloidal probe atomic force microscopy (AFM) [23] or interferometry [24] , [25] , are mostly limited to (sub)micrometer objects. The state-of-the-art of single-particle contact angle measurements is currently the gel-trapping technique (GTT) [26] , combined with scanning electron microscopy (SEM) for sub-micrometer colloids [26] or with AFM for NPs down to 74 nm (ref. 27 ). Despite its success, this approach presents several limitations. The choice of the liquid phases is limited owing to the high temperatures involved in the gel processing (close to the boiling point of important nonpolar phases such as n -hexane) and that changes to the aqueous phase, for example, ionic strength, affect the gelling. Also, the length scale of the gelling agent is comparable to the size of small NPs [28] , and therefore inhomogeneities in the trapping and measurements are expected to occur. GTT is moreover typically performed using a spreading solvent to ensure sufficient trapping on particle injection at the interface. Spreading solvents have been demonstrated to affect strongly the particle wetting properties, even turning particles form hydrophilic to hydrophobic [29] , [30] . Finally, AFM–GTT, because of tip convolution, is not able to measure simultaneously the radius and the height of the particles at the interface, and, therefore, single-particle contact angle measurements become impossible for nanoparticles and only averaged θ can be calculated by introducing NP size distributions. Here we present a novel method based on freeze-fracture shadow-casting (FreSCa) and cryo-SEM imaging that overcomes all the issues put forth above and pushes the limit of single-particle contact angle measurements down to NPs in the 10 nm diameter range. We successfully measured contact angles of hydrophilic and hydrophobic, organic and inorganic NPs, in-situ at the interface between water and different organic solvents. Our method allows for single-particle resolution and overcomes artefacts and limitations present in other techniques, as described further in the text. The high accuracy of the proposed approach makes it also possible to highlight significant heterogeneity in the wetting of NPs that has direct consequences on their adsorption and assembly at fluid interfaces. Single-particle contact angle determination by FreSCa cryo-SEM Freeze-fracture was originally developed for imaging protein and lipid nanostructures on cell membranes for biological structure determination [31] , and it has become the standard technique to characterize lipid–water interfaces of isolated systems [32] or within cells [33] . The proposed procedure is shown in Figure 1c : a particle-laden liquid–liquid interface is created, frozen and fractured exposing immobilized NPs that are then unidirectionally metal-coated at an oblique angle α. The interface acts as a weak fracture plane, and, therefore, it is preferentially exposed on fracturing ( Supplementary Fig. S1 ). The unidirectional metal deposition creates a shadow behind each of the features protruding from the interface. By measuring the shadow length k and the projected height l , and knowing the shadowing angle α, one can determine precisely the exposed height h of each feature. The case of spherical NPs of radius r is schematically represented in Figure 1a,b for hydrophilic and hydrophobic NPs, respectively. The individual contact angle θ can be directly obtained from the geometric relation θ= cos −1 ( |h-r|/r ). For spherical hydrophobic NPs, the particle equator is exposed, and, thus, its radius r is directly measurable, giving: For hydrophilic NPs, the particle equator lies below the ice surface, and a more complex set of geometrical relations between the measured quantities has to be used to obtain: (see Supplementary Note 1 for the full derivation). In both cases, we note that the calculated values of the contact angle depend only on the shadowing angle and on the measured ratios l/r and l/k , for hydrophobic and hydrophilic particles, respectively. 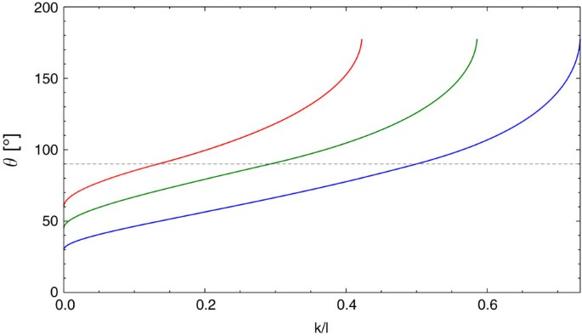Figure 2: Contact angle calculations from measured quantities. Values of contact anglesθcalculated according to equations (1) and (2) as a function ofk/lfor shadowing angles α=30° (blue), 45° (green) and 60° (red). For hydrophobic particles, equation (1) expressesθas a function ofl/rthat can be readily converted to the units of this graph given that, in this case,l–kcoincides with the actual particle radiusr. Increasing α leads to a smaller range of working parameters. Exploiting the fact that for hydrophobic particles r=l−k , the results of equations (1) and (2) can be plotted as a function of the measured parameter ratio k/l only, as shown in Figure 2 for α=30°, 45° and 60°. The attainable values of θ have an upper limit θ = π and a lower one set by geometry θ =α. By decreasing the shadowing angle, one is, therefore, able to measure increasingly hydrophilic particles. Moreover, we note that using shallower coating angles also increases the range of working parameters (that is, greater k/l range). As will be discussed later in the paper, changing α also influences the accuracy of the technique. Figure 2: Contact angle calculations from measured quantities. Values of contact angles θ calculated according to equations (1) and (2) as a function of k/l for shadowing angles α=30° (blue), 45° (green) and 60° (red). For hydrophobic particles, equation (1) expresses θ as a function of l/r that can be readily converted to the units of this graph given that, in this case, l–k coincides with the actual particle radius r . Increasing α leads to a smaller range of working parameters. 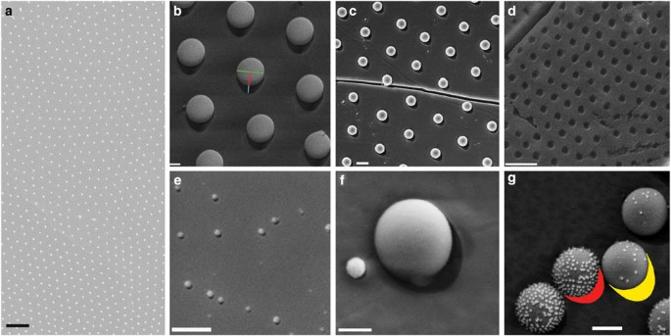Figure 3: Cryo-SEM images of different NPs at the liquid–liquid interface after freeze-fracture. The shadow cast by the nanoparticles (NPs) on metal deposition is visible in the high-magnification images. (a) Low-magnification image of 200 nm amidine latex particles at then-decane/water interface. Scale bar, 3 μm. (b) 500 nm amidine latex particles at then-decane/water interface. The key quantities necessary to measure the contact angle are highlighted for one particle: particle diameter (green), projected heightl(red+cyan) and shadow lengthk(cyan). Scale bar, 200 nm. (c) 200 nm amidine latex particles at the water/n-hexane interface. A further fracture line in the ice is visible. Scale bar, 300 nm. (d) Hollow prints left by 500 nm amidine latex particles in the frozenn-decane side of the interface. Scale bar, 2 μm. (e) 20 nm amidine latex particles at then-decane/water interface. Scale bar, 200 nm. (f) 100 nm hydrophilic citrate gold NP next to a 500 nm amidine latex NP at the water/n-decane interface. Scale bar, 200 nm. (g) 500 nm amidine latex NPs coated by 20 nm citrate gold NPs at the water/n-decane interface. Higher surface coverage of gold NPs renders the larger colloids more hydrophilic. Scale bar, 300 nm. Full size image Cryo-SEM images of NPs at fluid interfaces The success of our approach is demonstrated by the results shown in Figure 3 (further examples are found in Supplementary Figs S2-S6 ). At low magnification, the in-plane structure of the NP assembly can be investigated. As shown in Figure 3a , regular, non-close packed hexagonal arrays are found over large areas, as previously reported [14] , but earlier observations concerned either micrometer-sized objects [16] or NP-monolayers transferred onto solid substrates [13] , whereas we present here the first direct, in-situ observation of interfacial assemblies of NPs in the ≤10 2 nm range. At higher magnification the shadow behind each particle is clearly visible. Figure 3b shows 500 nm amidine polystyrene latex particles at a water/ n -decane interface; the dimensions necessary to measure θ are highlighted for one particle. Figure 3c shows 200 nm amidine polystyrene latex particles at the water/ n -hexane interface, demonstrating the success of the method for a solvent pair not accessible by GTT. The complete capture of NPs at the side of the frozen water and long-range ordering is also demonstrated by the prints left by 500 nm particles in the frozen n -decane ( Fig. 3d ). The most important result consists in the measurement of contact angles of very small NPs, as highlighted in Figure 3e ; an image of 20 nm amidine polystyrene latex NPs at the water/ n -hexane interface is shown, where the shadow of individual particles can be measured at high magnification. The smallest measured particle had a radius of 4.7 nm, which pushes the limits of single-particle contact angle measurements down by almost two orders of magnitude down. Figure 3f also shows the capability of the method to measure hydrophilic particles, namely 100 nm citrate gold NPs at the water/ n -decane interface. Finally, Figure 3g highlights the possibility of measuring variations in contact angle resulting from chemical or topological modifications to the particle surface within a particle batch. The contact angles of 500 nm hydrophobic amidine latex colloids coated by 20 nm hydrophilic citrate gold NPs at the water/ n -decane interface were measured, and, for a higher Au NP coverage, a reduction in the contact angle was found. Figure 3: Cryo-SEM images of different NPs at the liquid–liquid interface after freeze-fracture. The shadow cast by the nanoparticles (NPs) on metal deposition is visible in the high-magnification images. ( a ) Low-magnification image of 200 nm amidine latex particles at the n -decane/water interface. Scale bar, 3 μm. ( b ) 500 nm amidine latex particles at the n -decane/water interface. The key quantities necessary to measure the contact angle are highlighted for one particle: particle diameter (green), projected height l (red+cyan) and shadow length k (cyan). Scale bar, 200 nm. ( c ) 200 nm amidine latex particles at the water/ n -hexane interface. A further fracture line in the ice is visible. Scale bar, 300 nm. ( d ) Hollow prints left by 500 nm amidine latex particles in the frozen n -decane side of the interface. Scale bar, 2 μm. ( e ) 20 nm amidine latex particles at the n -decane/water interface. Scale bar, 200 nm. ( f ) 100 nm hydrophilic citrate gold NP next to a 500 nm amidine latex NP at the water/ n -decane interface. Scale bar, 200 nm. ( g ) 500 nm amidine latex NPs coated by 20 nm citrate gold NPs at the water/ n -decane interface. Higher surface coverage of gold NPs renders the larger colloids more hydrophilic. Scale bar, 300 nm. Full size image Accuracy of FreSCa cryo-SEM contact angle measurements Our method yields unprecedented single-particle accuracy, allowing for characterization of individual particles that can disclose new aspects of micro- and nano-particle wetting. The accuracy σ θ in measuring contact angles as a function of the measured quantities can be directly derived from equations (1) and (2) to yield for hydrophobic particles and for hydrophilic particles, where σ l , σ r , and σ k are the accuracies in the measured quantities l , r , and k (see Supplementary Note 2 for the full derivation). The limiting factor in measuring accurately the particle dimensions and the shadow lengths in the SEM images is the pixel size relative to the object size. From sharp SEM images, we can measure features with±1 pixel accuracy ( σ l and σ k =1 pixel, σ r =0.5 pixel because the particle diameter is actually measured). This means that, regardless of the magnification used, particles with a diameter and a shadow length smaller than 3 pixels are discarded as being not resolvable; in practice, we never imaged particles with a radius and a shadow length below 5 pixels. From equations (3) and (4), it is apparent that reducing the relative error in measuring l , r , and k increases the measurement accuracy. As σ l , σ r and σ k are fixed, a higher accuracy can be achieved by increasing the size of the measured features, that is, by working at higher magnification and/or using a higher image resolution. The highest achieved image resolution was 0.7 nm per pixel (after 20 s dwell time per image averaging). Another option is to lower the shadowing angle; shallower-coating angles cast longer shadows, reducing the errors in measuring l and k . 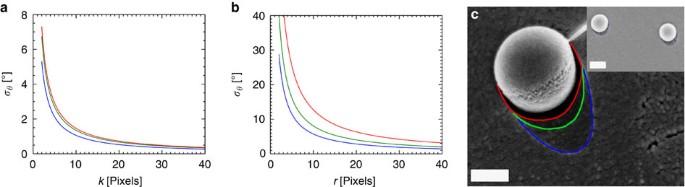Figure 4: Accuracy of FreSCa cryo-SEM contact angle measurements. (a) Error in contact angle measurementsσθby FreSCa calculated according to equations (3) and (4) as a function ofkfor fixedk/l=0.1 for shadowing angles α=30° (blue), 45° (green) and 60° (red), corresponding, respectively, to contact angles of 46°, 67° and 85°. Any other choice ofk/lleads to the same qualitative behaviour.σθdecreases for increasingkand with smaller shadowing angles. (b)σθas a function ofrfor a fixed contact angleθ=110° for shadowing angles α=30° (blue), 45° (green) and 60° (red). The accuracy is increased by reducing α and for larger particles. Any other choice ofθleads to equivalent results. (c) Cryo-SEM image of a 500 nm amidine latex nanoparticle (NP) at the frozen water/n-decane interface. The sample was coated three times in succession with 3 nm of tungsten, each time at a different shadowing angle to produce shadows of different lengths as highlighted on the image: α=30° (blue), α=45° (green) and α=60° (red). The graininess of the background and of the particle surface is due to the thick metal layer from to the triple coating. Inset: cryo-SEM image of two neighbouring 200 nm amidine latex NPs at the frozen water/n-decane interface. Despite having the same size, the two particles show significantly different contact angles (left particler=116.4±2.5 nmθ=96.9±3.13°; right particler=116.3±2.5 nmθ=102.0±3.24°), highlighting the heterogeneity of wetting on the nanoscale. Scale bars, 200 nm. These results are more clearly presented in Figure 4 . Figure 4a shows σ σ as a function of k for a fixed ratio k/l =0.1 for α=30°, 45° and 60°; any other choice of k/l shows the same behaviour. It is evident from the graph that for the same values of the measured parameter ratio k/l (which determines the contact angle) larger values of k lead to higher accuracy. Additionally, σ θ is also reduced for lower α. Similarly, when fixing the contact angle (that is, 110° in this case), we note again the same behaviour in terms α and magnitude of the measured quantity r (see Fig. 4b ). The largest actual error in our measured data was 16.3° for a particle with contact angle 119.30° and radius 6.67 nm; the contact angles of all the other imaged particles were measured with significantly higher accuracy. Table 1 reports the average error for each data set measured. Figure 4: Accuracy of FreSCa cryo-SEM contact angle measurements. ( a ) Error in contact angle measurements σ θ by FreSCa calculated according to equations (3) and (4) as a function of k for fixed k/l =0.1 for shadowing angles α=30° (blue), 45° (green) and 60° (red), corresponding, respectively, to contact angles of 46°, 67° and 85°. Any other choice of k/l leads to the same qualitative behaviour. σ θ decreases for increasing k and with smaller shadowing angles. ( b ) σ θ as a function of r for a fixed contact angle θ =110° for shadowing angles α=30° (blue), 45° (green) and 60° (red). The accuracy is increased by reducing α and for larger particles. Any other choice of θ leads to equivalent results. ( c ) Cryo-SEM image of a 500 nm amidine latex nanoparticle (NP) at the frozen water/ n -decane interface. The sample was coated three times in succession with 3 nm of tungsten, each time at a different shadowing angle to produce shadows of different lengths as highlighted on the image: α=30° (blue), α=45° (green) and α=60° (red). The graininess of the background and of the particle surface is due to the thick metal layer from to the triple coating. Inset: cryo-SEM image of two neighbouring 200 nm amidine latex NPs at the frozen water/ n -decane interface. Despite having the same size, the two particles show significantly different contact angles (left particle r =116.4±2.5 nm θ =96.9±3.13°; right particle r =116.3±2.5 nm θ =102.0±3.24°), highlighting the heterogeneity of wetting on the nanoscale. Scale bars, 200 nm. Full size image Table 1 Summary of measured quantities. Full size table To explore further the effect of changing α, we performed an experiment where 500 nm amidine latex particles frozen at the water/ n -decane interface were coated in succession at 30°, 45° and 60°. An example of the obtained results is reported in Figure 4c displaying three distinct shadows behind the imaged particle corresponding to the different coating angles. From the measured quantities, we can calculate θ =96.21±1.91°, 95.89±2.80° and 97.75±4.55° for α=30°, 45° and 60°, respectively. Again we observe that increasing the coating angle increases the error. All the data reported further have been collected with α=45°. Contact angle distributions Figures 5 and 6 report contact angle distributions for different particle materials, surface chemistry, sizes and liquid phases. 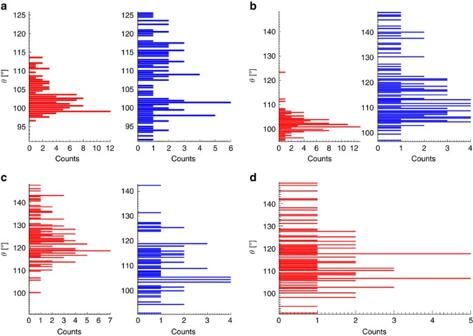Figure 5: Distribution of measured contact angles for individual nanoparticles. (a) 500 nm amidine latex at the water/n-decane (red) and water/n-hexane (blue) interface. (b) 200 nm amidine latex at the water/n-decane (red) and water/n-hexane (blue) interface. (c) 100 nm amidine (red) and sulphate (blue) latex at the water/n-decane. (d) 40 nm amidine latex at the water/n-decane interface. In Figure 5a,b, the effect of switching the nonpolar phase between n -decane and n -hexane is highlighted for 500 and 200 nm particles, respectively. For the latter solvent, much broader θ distributions are found, probably due to chemical degradation at the interface. Figure 5c shows instead the effect of changing the surface chemistry from amidine to sulphate terminated polystyrene latex for 100 nm NPs at the water/ n -decane interface, with the latter being more hydrophilic. The results for 40 nm amidine latex particles at the water/ n -decane interface are reported in Figure 5d . 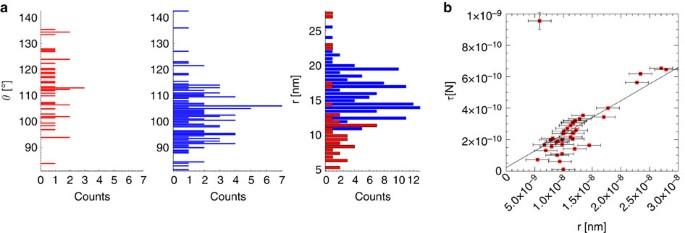Figure 6: Contact angle and line tension. (a) Distributions of measured contact angles for individual, nominally 20 nm amidine latex nanoparticles (from the same synthesis batch) and corresponding measured size distributions at the water/n-decane (red) and water/n-hexane (blue) interface. Note that the smallest particles are 10 nm in diameter. (b) Line tensionτas a function of radiusrfor 20 nm for the amidine latex particles at the water/n-decane interface. The solid line is a linear fit. The x-errors stem from the limits to the image resolution in measuringr(1 pixel); the errors inτare calculated according to equation (S22) in theSupplementary Note 4and are typically smaller than the symbols. The data for the smallest NPs, nominally 20 nm amidine latex particles from the same synthesis batch, at the n -decane and n -hexane/water interfaces, are shown in Figure 6a, where the contact angle distributions are accompanied by the measured size distributions at the interface. We observe that single-particle contact angles can be measured for NPs as small as 10 nm in diameter. The difference in the measured size distributions reflects the limitations in resolving particles below a given size in pixels. In fact for the water/ n -decane, we achieved the highest resolution (0.7 nm per pixel) whereas, for the n -hexane interface, the image resolution was limited to 1.2 nm per pixel, determining a higher cut-off in the resolvable particle size. Moreover, as previously discussed, longer shadows are cast for increasingly hydrophobic particles; this means that close to the resolution limit, the method produces contact angle distributions biased towards higher values, because more hydrophilic particles are discarded as not resolvable. The average values and standard deviations of the data in the figures are reported in Table 1 . Figure 5: Distribution of measured contact angles for individual nanoparticles. ( a ) 500 nm amidine latex at the water/ n -decane (red) and water/ n -hexane (blue) interface. ( b ) 200 nm amidine latex at the water/ n -decane (red) and water/ n -hexane (blue) interface. ( c ) 100 nm amidine (red) and sulphate (blue) latex at the water/ n -decane. ( d ) 40 nm amidine latex at the water/ n -decane interface. Full size image Figure 6: Contact angle and line tension. ( a ) Distributions of measured contact angles for individual, nominally 20 nm amidine latex nanoparticles (from the same synthesis batch) and corresponding measured size distributions at the water/ n -decane (red) and water/ n -hexane (blue) interface. Note that the smallest particles are 10 nm in diameter. ( b ) Line tension τ as a function of radius r for 20 nm for the amidine latex particles at the water/ n -decane interface. The solid line is a linear fit. The x-errors stem from the limits to the image resolution in measuring r (1 pixel); the errors in τ are calculated according to equation (S22) in the Supplementary Note 4 and are typically smaller than the symbols. Full size image Comparison with gel-trapping technique Finally, we make a direct comparison between our method and AFM–GTT for particles in the micrometer range, for which the latter offers single-particle resolution with accuracy comparable to the one of FreSCa cryo-SEM. 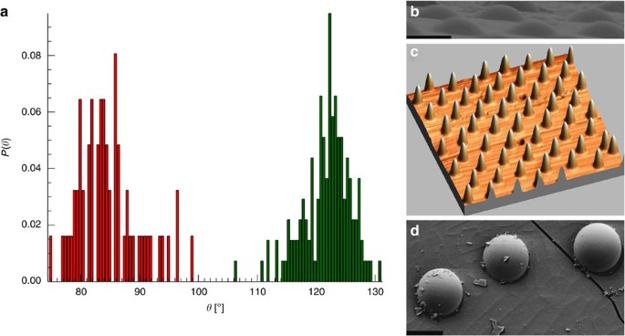Figure 7: Comparison with GTT. (a) Contact angle probability distributions P(θ) for 2.8 μm diameter polystyrene (PS) particles at the water/n-decane interfaces measured using FreSCa cryo-SEM (red) and AFM-GTT (green). The latter was performed in the presence of isopropanol as a spreading solvent that makes the colloids more hydrophobic. The average error in the individual data points is of 3.5° and 3.6° for the FreSCa cryo-SEM and the AFM–GTT respectively. (b) SEM image of the polystyrene (PS) particles embedded into the PDMS. The exposed part was originally immersed in the water phase. Scale bar, 2 μm. (c) AFM image of the PS particle protruding from the PDMS surface. The long-range order at the interface reflects the typical behaviour of hydrophobic particles. Lateral scan size 50 μm. The z-scale has been expanded for clarity; maximum particle height in the image: 958 nm. (d) Cryo-SEM image of 2.8 μm PS particles at the water/n-decane interface. The short shadows demonstrate the particle hydrophilicity. Scale bar, 2 μm. Figure 7 shows an example for 2.8 μm diameter polystyrene particles at the water/ n -decane interface. Both techniques have a resolution in the 3°–4° range for this system; for the AFM–GTT data, the main source of inaccuracy is the lateral resolution of the images (pixel size), whereas the particle height at the interface is measured with high precision ( Supplementary Note 3 ). It is evident that the contact angles measured with the two techniques are significantly different. This is to be ascribed to the use of a spreading solvent for the GTT; particles are injected and spread at the interface in a 0.4 wt% 4:6 isopropanol-water suspension [39] . As recently demonstrated [29] , [30] , the use of a spreading solvent has a strong influence on the measured wetting properties, with isopropanol making microparticles more hydrophobic. The hydrophobic character of the particles is evident from the SEM in Figure 7b , where we observe that the portion of the particles protruding from the polydimethylsiloxane (PDMS) surface (that is, the portion of the particles initially immersed in the water) is smaller than half the particles. Moreover, the long-range order at the interface (AFM image in Fig. 7c ), as typically observed for hydrophobic particles [16] , [40] , substantiates our observations in the presence of isopropanol. FreSCa has the advantage of not requiring the use of spreading agents. In this case, the particles are slightly hydrophilic ( Fig. 7d ). Despite the difference in the average values of the measured contact angles due to the presence of a spreading solvent, both techniques highlight a spread in the contact angles that is larger than the error in the individual data points, confirming further the heterogeneity of wetting for micro and nanoparticles. The width of the θ distribution is consistent between the two data sets. The quantitative comparisons with AFM–GTT for this system as well as for two extra ones are reported in Table 1 . Figure 7: Comparison with GTT. ( a ) Contact angle probability distributions P( θ ) for 2.8 μm diameter polystyrene (PS) particles at the water/ n -decane interfaces measured using FreSCa cryo-SEM (red) and AFM-GTT (green). The latter was performed in the presence of isopropanol as a spreading solvent that makes the colloids more hydrophobic. The average error in the individual data points is of 3.5° and 3.6° for the FreSCa cryo-SEM and the AFM–GTT respectively. ( b ) SEM image of the polystyrene (PS) particles embedded into the PDMS. The exposed part was originally immersed in the water phase. Scale bar, 2 μm. ( c ) AFM image of the PS particle protruding from the PDMS surface. The long-range order at the interface reflects the typical behaviour of hydrophobic particles. Lateral scan size 50 μm. The z-scale has been expanded for clarity; maximum particle height in the image: 958 nm. ( d ) Cryo-SEM image of 2.8 μm PS particles at the water/ n -decane interface. The short shadows demonstrate the particle hydrophilicity. Scale bar, 2 μm. Full size image The key result that can be extracted from the data presented in Figures 5 and 6 and summarized in Table 1 is that the spread in the contact angle distributions is greater than the error in the single-particle measurement, highlighting the fact that the wide distributions are not due limitations in the resolution of the method for the contact angle measurement. Large-scale heterogeneity of the interface could be the cause of the broad distributions, but contact angles measured on different samples as well as on the same interface on mm 2 scales showed no systematic variations. Moreover, the inset to Figure 4c highlights the fact that two neighbouring 200 nm amidine latex particles of identical size show significantly different contact angles, underlining the fact that the heterogeneity of the wetting properties probably derives from the distribution of surface properties of the nanoscale materials themselves. Broadening of θ distributions at the nanoscale can also stem from the presence of Brownian motion. NPs are trapped at the interface with an energy Δ E , as discussed previously, but, for small objects, thermal motion can be significant enough to displace them from their individual equilibrium position relative to the interface. The FreSCa method takes a snapshot of the particles at the interface and therefore intrinsically a distribution of heights (and thus of contact angles) is measured. As reported in the literature, the shape of the potential well around the equilibrium position at the interface is quadratic with the displacement [11] , [14] , [15] , and the probability distribution of finding a particle at position z from the bottom of the well will be proportional to . Using the full expression for Δ E(z) and neglecting line tension contributions [11] , the width of the z -displacement distribution is , where . For the smallest investigated particles with r =5 nm particle at the water/ n -decane interface, this corresponds to a width of the displacement distribution of 2.6% of the particle radius that translates into a±3° error in measuring θ for a NP with an equilibrium contact angle of 150°, which is significantly smaller than the observed distribution width. For larger particles, this effect becomes rapidly negligible. Polydispersity for small nanoparticles can also introduce further spreading of the contact angle distributions due to line tension effects. In fact, line tension contributions to θ depend on particle size and become increasingly more relevant at the nanoscale [15] . The unprecedented resolution of our method allows for measuring directly the line tension of individual NPs. Figure 6b shows the values of the line tension τ vs. r for the nominally 20 nm particles at the water/ n -decane interface; our data indeed follow a linear scaling with the size as from theoretical predictions [15] and the values we measured are consistent with previous findings [11] (more details in the Supplementary Note 4 ). Summarizing, broad θ distributions are found for the same NP material, with increasing spread of the contact angle values for smaller NPs. For the reasons discussed above, this reflects the fact that the wetting behaviour of colloidal particles becomes heterogeneous at the micro- and nano-scale where the details of surface properties (for example, chemistry, shape and topography) make relatively larger contributions to the average bulk material properties. For instance, as recently demonstrated, interparticle interactions at liquid interfaces strongly depend on the individual particles chosen for the measurement [34] . This demonstrates the need for true single-particle characterization that has already been undertaken by numerical simulations [35] , [36] , [37] , [38] but up to now has been missing experimentally. In conclusion, we have described a new characterization method on the basis of freeze-fracture and shadow-casting cryo-SEM that enabled us to measure directly for the first time three-phase contact angles in-situ at diverse water–oil interfaces for individual nanoparticles as small as 10 nm. Our technique places itself at the forefront of the currently available characterization methods in terms of capability, resolution and flexibility. Key fundamental questions, including line tension, surface roughness and homogeneity of surface chemistry, demand characterization of wetting properties on the single-NP level that can be met by this technique. Finally, we foresee the extension of our approach to the investigation of interfacial assembly and wetting properties of many more systems, including anisotropic particles, for which orientation at the interface can be directly measured with our technique, and composite, core-shell nanoparticles. This will help improve the current basic understanding and applications of NPs for which interfacial control is essential. Materials Amidine polystyrene latex, sulphate polystyrene latex nanoparticles were from Invitrogen/Interfacial Dynamics and citrate gold nanoparticles from BBI International. We additionally used, for the comparison with AFM–GTT, polystyrene particles from Microparticles GmBH, and poly(methyl methacrylate) (PMMA) particles synthesized in-house and kindly provided by Dr. A. Schofield. The particle sizes are found in the Supplementary Tables S1, S2 and S3 . Particle solutions were diluted or concentrated by centrifugation in MilliQ water ( R =18.2 Ω, TAC<6 p.p.b.) and ultrasonicated for several minutes, with the exception of the PMMA particles that were dispersed in n -decane. n -hexane (Ultra Violet spectroscopy grade, Sigma-Aldrich) and n -decane (≥99%, Aldrich-Fine Chemicals) were used as delivered. Freeze-fracture and metal coating 0.5 μl of an aqueous NP suspension were placed inside a custom-made copper holder with a 200 μm deep central cavity ( Supplementary Fig. S9 ). Before use, the sample holders were cleaned in sulphuric acid 95% and ethanol for several minutes, and their inner surface was roughened to improve adhesion during freezing. Successively, a 3.0 μl droplet of the nonpolar phase was carefully placed on top to create the liquid–liquid interface, and then the holder was closed with a flat copper plate. The 'sandwich' holder was frozen in a liquid propane jet freezer (Bal-Tec/Leica JFD 030) with a cooling rate of 30 000 Ks −1 to avoid water crystallization. After freezing, the samples were mounted under liquid nitrogen onto a double fracture cryo-stage and transferred under inert gas in a cryo-high vacuum airlock (<5×10 −7 mbar Bal-Tec/Leica VCT010) to a pre-cooled freeze-fracture device at −140°C (Bal-Tec/Leica BAF060 device). The samples were then fractured and partially freeze-dried at −110°C for 3 min to remove deposited residual water condensation and ice crystals, followed by unidirectional tungsten deposition at an elevation angle α=45° to a total thickness δ =2 nm at −120°C and by extra 2 nm with a continuously varying angle between 90° and 45°. The second deposition is needed to avoid charging of the shadow during imaging that may compromise image stability at high magnifications. Cryo-SEM imaging Freeze-fractured and metal-coated samples were then transferred for imaging under high vacuum (<5×10 −7 mbar) at −120°C to a pre-cooled (−120°C) cryo-SEM (Zeiss Gemini 1530) for imaging either with an in-lens or secondary electron detector. How to cite this article: Isa L. et al . Measuring single-nanoparticle wetting properties by freeze-fracture shadow-casting cryo-scanning electron microscopy. Nat. Commun. 2:438 doi: 10.1038/ncomms1441 (2011).